Plexin-A4-dependent retrograde semaphorin 3A signalling regulates the dendritic localization of GluA2-containing AMPA receptors The dendritic targeting of neurotransmitter receptors is vital for dendritic development and function. However, how such localization is established remains unclear. Here we show that semaphorin 3A (Sema3A) signalling at the axonal growth cone is propagated towards the cell body by retrograde axonal transport and drives AMPA receptor GluA2 to the distal dendrites, which regulates dendritic development. Sema3A enhances glutamate receptor interacting protein 1-dependent localization of GluA2 in dendrites, which is blocked by knockdown of cytoplasmic dynein heavy chain. PlexinA (PlexA), a receptor component for Sema3A, interacts with GluA2 at the immunoglobulin-like Plexin-transcription-factor domain (PlexA-IPT) in somatodendritic regions. Overexpression of PlexA-IPT suppresses dendritic localization of GluA2 and induces aproximal bifurcation phenotype in the apical dendrites of CA1 hippocampal neurons. Thus, we propose a control mechanism by which retrograde Sema3A signalling regulates the glutamate receptor localization through trafficking of cis-interacting PlexA with GluA2 along dendrites. Neurons are compartmentalized into two molecularly and functionally distinct domains, axons and dendrites. The precise targeting and localization of proteins within these domains is critical for every aspect of neuronal function. α-Amino-3-hydroxy-5-methylisoxazole-4-propionic acid (AMPA)-type glutamate receptors are composed of heteromeric combinations of GluA1 to GluA4 (ref. 1 ) and are the major excitatory neurotransmitter receptors in the central nervous system. The diversity in regulation of AMPA receptor subunit expression suggests that changes in the properties of AMPA receptors serve specific functions in a variety of brain areas. Altering the level of AMPA receptor activity has also been shown to play an important role in dendritic patterning and synapse maturation and formation [2] , [3] , and disturbance of AMPA receptor localization has been implicated in many psychiatric and neurological disorders [4] . The dendritic targeting of AMPA receptors is therefore a crucial part of dendritic development and function. However, little is known about how extrinsic molecules regulate the dendritic localization of AMPA receptors. AMPA receptor localization can be regulated by some axon guidance molecules, which act as short-range synaptogenic factors. For example, ephrins-to-EphB forward signalling controls excitatory synapses, and reverse EphB2 signalling from postsynaptic sites triggers presynaptic differentiation through ephrin binding [5] . UNC-6/netrin also mediates adhesive interactions to promote synaptogenesis [6] . Semaphorin 3A (Sema3A) is a secreted protein identified as a factor that collapses and paralyses the neuronal growth cone by acting on a growth cone receptor complex of neuropilin1 (NRP1) and plexinAs (PlexAs) [7] , [8] , [9] , [10] . Sema3A has multiple functions in the regulation of both axonal and dendritic development. Disruption of Sema3A in mice leads to axonal sprouting of several cranial nerves, distortion of odour maps in the olfactory bulb, disorientation of apical dendrites of large pyramidal cells and insufficient maturation of dendritic spines in the cerebral cortex [11] , [12] , [13] , [14] , [15] , [16] , [17] , [18] , [19] . In this study, using hippocampal neurons at early developmental axon outgrowth stage [20] , we investigate the role of Sema3A in dendritic targeting of AMPA receptors. Based on in vivo and in vitro data, we demonstrate that local signalling of Sema3A at the axonal growth cone induces a retrograde axonal transport of PlexA4, which in turn regulates the localization of AMPA receptor subunit GluA2 in dendrites, contributing the dendritic development. Our findings reveal a novel mechanism of dendritic AMPA receptor localization, in which PlexA4 mediates growth cone Sema3A signalling and acts as a cis-interacting receptor with GluA2 in somatodendritic regions, escorting GluA2 to the distal dendrites. Sema3A at distal axon induces dendritic GluA2/3 localization Using time-lapse video microscopy, we previously demonstrated that Sema3A facilitates organelle transport along axon of dorsal root ganglion (DRG) neurons, pseudounipolar neurons that contain an axon splitting into two branches [21] . Sema3A transiently facilitates the percentage of moving particles, and these particles monitored by time-lapse video microscopy are composed mainly of mitochondria and non-mitochondrial particles [10] , [21] . The transported particles observed generally have maximal diameters of >0.2 μm, and the velocity of these moving particles ranges from 0.6 to 4.5 μm s −1 in both antero- and retrograde transport. The velocity of moving particles suggests that the transport involved is a fast microtubule-dependent trafficking event [21] . To examine whether the effect of Sema3A is also observed in dendrites, stage 3 cultured hippocampal neurons, at an early stage of 3 days in vitro (3DIV) culture of neurons from embryonic day 18 (E18) rat embryos, in which a single prominent axon can be easily distinguished from several short dendrites [20] , were used to analyse the rate of transport in both axon and dendrite ( Supplementary Fig. 1a ). Bath application of Sema3A (5 nM) to hippocampal neurons facilitated dendritic transport as well as axonal transport. A polarized response to Sema3A was also observed: local application of Sema3A to the axonal growth cone, but not to the axonal shaft, soma or dendritic growth cone, facilitated both axonal and dendritic transport ( Supplementary Fig. 1b,c ), suggesting that Sema3A-induced signal is propagated from axon to somatodendrite. We next examined the possible cargo proteins involve in the Sema3A-induced facilitation of dendritic transport. Because Sema3A has been shown to induce dendritic maturation [13] , [17] , we performed immunocytochemical analysis of several ionotropic glutamate receptor subunits in 3DIV hippocampal neurons. The time of fixation was set to be 30 min after the Sema3A treatment because the effect of facilitated axonal and dendritic transport returned to the basal level after 30 min ( Supplementary Fig. 1b ). Sema3A enhanced the immunostaining of GluA2 in MAP2-positive dendrites (control: 100.0±3.2%, n =50; Sema3A: 191.3±14.0%, n =50, P <0.01 by t -test). Sema3A did not change the levels of GluA1 (control: 100.0±4.5%, n =30; Sema3A: 98.5±3.3%, n =30, P >0.05 by t -test) and GluN1 (control: 100.0±3.7%, n =30; Sema3A: 105.5±5.1%, n =30, P >0.05 by t -test), a subunit of N -methyl- D -aspartate receptors ( Fig. 1a ). The enhanced expression levels of GluA2 was still observed in dendrites of non-permeabilized neurons (control: 100.0±5.0%, n =45; Sema3A: 141.8±8.6%, n =45, P <0.01 by t -test; Fig. 1a ), suggesting that Sema3A increases the surface expression of GluA2. In hippocampus, most AMPA receptors are heterotetramers composed of GluA1/GluA2 or GluA2/GluA3 (ref. 22 ). Sema3A also enhanced the immunostaining of GluA3 in dendrites (control: 100.0±1.6%, n =30; Sema3A: 124.0±3.7%, n =30, P <0.01 by t -test; Fig. 1a ). This finding indicates that Sema3A induced the dendritic localization of GluA2/3 heterotetramers. 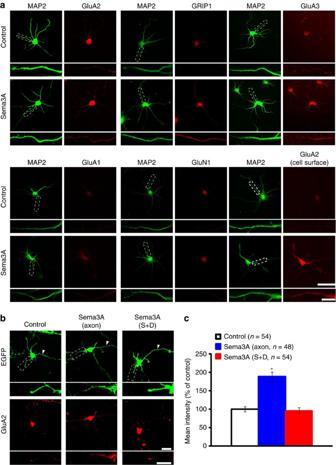Figure 1: Sema3A enhances immunostaining of GluA2/3 and GRIP1 in dendrites. (a) Sema3A enhanced immunostaining of GluA2, GluA3 and GRIP1 without modifying those of GluA1 and GluN1 in the MAP2-positive dendrites of cultured hippocampal neurons. Sema3A also enhanced expression levels of GluA2 in the cell surface of dendrites. (b) Sema3A applied at the axonal region, but not somatodendritic region (S+D), enhanced immunostaining of GluA2 in the dendrites of cultured hippocampal neurons. Representative images of the somatodendritic regions (indicated in the box inSupplementary Fig. 1e) are shown. Arrowheads inbindicate axon. Normalized mean immunostaining intensity of dendrite per neuron is shown inc(n=48–54 neurons from more than three independent cultures). Magnified images of boxed areas in upper panels are shown in lower panels (aandb). Scale bars ina, 50 μm (upper panel); 10 μm (lower panel);b, 20 μm (upper panel) or 10 μm (lower panel). *P<0.01 by ANOVA compared with vehicle control. Data are presented as mean±s.e.m. Figure 1: Sema3A enhances immunostaining of GluA2/3 and GRIP1 in dendrites. ( a ) Sema3A enhanced immunostaining of GluA2, GluA3 and GRIP1 without modifying those of GluA1 and GluN1 in the MAP2-positive dendrites of cultured hippocampal neurons. Sema3A also enhanced expression levels of GluA2 in the cell surface of dendrites. ( b ) Sema3A applied at the axonal region, but not somatodendritic region (S+D), enhanced immunostaining of GluA2 in the dendrites of cultured hippocampal neurons. Representative images of the somatodendritic regions (indicated in the box in Supplementary Fig. 1e ) are shown. Arrowheads in b indicate axon. Normalized mean immunostaining intensity of dendrite per neuron is shown in c ( n =48–54 neurons from more than three independent cultures). Magnified images of boxed areas in upper panels are shown in lower panels ( a and b ). Scale bars in a , 50 μm (upper panel); 10 μm (lower panel); b , 20 μm (upper panel) or 10 μm (lower panel). * P <0.01 by ANOVA compared with vehicle control. Data are presented as mean±s.e.m. Full size image To determine the site of Sema3A action, we employed the microfluidic culture system, which enabled us to perform local stimulation to the axonal or somatodendritic region by isolating these two parts ( Supplementary Fig. 1d,e ) [23] . Sema3A when locally applied to the axonal areas (188.1±12.8%, n =48), but not somatodendritic areas (95.9±8.7%, n =54), increased the immunostaining of GluA2 in the dendrites ( Fig. 1b,c ). This finding suggests that Sema3A signalling propagates from the axonal growth cone and induces the dendritic localization of GluA2. Sema3A drives GRIP1 and GluA2 to dendrites GluA2 is transported from the cell body to dendrite by the glutamate receptor interacting protein 1 (GRIP1)/kinesin superfamily protein 5 (KIF5) complex [24] . GRIP1 is a neuronal scaffolding protein that interacts directly with the C termini of GluA2/3 but not GluA1 (ref. 25 ). If the transport of GluA2 is involved in the dendritic localization of GluA2, then Sema3A may also increase GRIP1 immunostaining signals in the dendrites. In cultured hippocampal neurons, Sema3A enhanced the immunostaining intensity of GRIP1 (control: 100.0±3.7%, n =30; Sema3A: 131.7±7.8%, n =30, P <0.01 by t -test; Fig. 1a ). To further determine the role of GRIP1, we performed siRNA knockdown of GRIP1 (ref. 26 ). Sema3A-enhanced immunostaining of GluA2 was markedly attenuated in neurons transfected with GRIP1-siRNA plasmid (107.6±6.5%, n =50), in which GRIP1 expression was suppressed ( Fig. 2a,b ; Supplementary Fig. 2a,c ). This attenuation was rescued by expressing a siRNA-resistant form of GRIP1 (154.0±7.4%, n =44; Fig. 2a,b ; Supplementary Fig. 2b,d ). Because knockdown of GRIP1 inhibits dendrite morphogenesis in mature neurons [26] , it is possible that the impaired dendrite development might be an indirect cause of the failure of GluA2 recruitment. However, the mean length of neurites was not affected by GRIP1 knockdown (control: 43.0±1.72 μm, n =74; knockdown: 47.4±1.9 μm, n =64, P >0.05 by t -test) in 3DIV hippocampal neurons. In addition, overexpression of KIF5-dominant negative (DN) mutant (KHCCBD) that contains the GRIP1-binding site, but lacks the kinesin light chain-binding site [24] , attenuated Sema3A-enhanced immunostaining of GluA2 (83.5±4.4%, n =30; Fig. 2c,d ). These findings suggest that Sema3A enhances the transport of GluA2 and localized the receptor to dendrites. 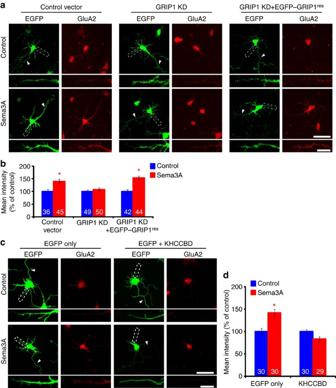Figure 2: Sema3A induces dendritic localization of GluA2 in a GRIP1- and KIF5-dependent manner. (a) Knockdown of GRIP1 attenuated Sema3A-enhanced immunostaining of GluA2 in dendrites. This attenuation was rescued by expressing a siRNA-resistant form of EGFP-GRIP1 (GRIP1res). Normalized mean immunostaining intensity of dendrite per neuron is shown inb(n=36–50 neurons from more than three independent cultures). (c) Overexpression of KIF5 DN mutant (KHCCBD) attenuated Sema3A-enhanced immunostaining of GluA2 in dendrites. Normalized mean immunostaining intensity of dendrite per neuron is shown ind(n=29–30 neurons from three independent cultures). Magnified images of boxed areas in upper panels are shown in lower panels. Arrowheads indicate axon. Scale bars, 50 μm (upper panel);10 μm (lower panel). *P<0.01 by ANOVA compared with vehicle control. Data are presented as mean±s.e.m. Figure 2: Sema3A induces dendritic localization of GluA2 in a GRIP1- and KIF5-dependent manner. ( a ) Knockdown of GRIP1 attenuated Sema3A-enhanced immunostaining of GluA2 in dendrites. This attenuation was rescued by expressing a siRNA-resistant form of EGFP-GRIP1 (GRIP1 res ). Normalized mean immunostaining intensity of dendrite per neuron is shown in b ( n =36–50 neurons from more than three independent cultures). ( c ) Overexpression of KIF5 DN mutant (KHCCBD) attenuated Sema3A-enhanced immunostaining of GluA2 in dendrites. Normalized mean immunostaining intensity of dendrite per neuron is shown in d ( n =29–30 neurons from three independent cultures). Magnified images of boxed areas in upper panels are shown in lower panels. Arrowheads indicate axon. Scale bars, 50 μm (upper panel);10 μm (lower panel). * P <0.01 by ANOVA compared with vehicle control. Data are presented as mean±s.e.m. Full size image The dendritic transport of GRIP1 was monitored by fluorescence recovery after photobleaching (FRAP) analysis of enhanced green fluorescent protein (EGFP)-tagged GRIP1. We examined the effect of Sema3A on fluorescence recovery of the ratio of EGFP-GRIP1 to mcherry in the photobleached dendrites from 7 to 11 min after Sema3A stimulation, when the peak effect of Sema3A on dendritic transport monitored by time-lapse video microscopy was seen ( Supplementary Fig. 1b ). Bath application of Sema3A enhanced the fluorescence recovery of EGFP-GRIP1 ( Fig. 3a–c ). Furthermore, local application of Sema3A at axonal growth cone, but not dendritic growth cone, enhanced the fluorescence recovery ( Fig. 3d,e ), consistent with the enhanced immunostaining of GluA2 in dendrites ( Fig. 1b,c ). We could not observe the transport of EGFP-GluA2 after FRAP in dendrites at 3DIV. Most of the over-expressed EGFP-GluA2 at 3DIV was probably localized at cell surface, because the EGFP-GluA2 fluorescent signals were almost completely quenched by bromophenol blue (BPB), a membrane-impermeable reagent that quenches the fluorescence of extracellularly exposed EGFP on the surface ( Supplementary Fig. 3a ) [27] . At a later stage of 6DIV, Sema3A was still able to induce dendritic localization of GluA2 (see below). We then attempted to obtain quantitative data from FRAP analysis in neurons at 6DIV. At this stage, the fluorescent signals of EGFP-GluA2 in dendrites were also quenched by BPB, but some fluorescence signals were resistant to BPB ( Supplementary Fig. 3a ). Under this condition, Sema3A enhanced fluorescence recovery of EGFP-GluA2 within the photobleached area ( Fig. 3f–h ). Taken together, our results provide evidence that a retrograde Sema3A signalling from axonal growth cone enhances GRIP1- and KIF5-dependent anterograde dendritic transport of GluA2, leading to the upregulation of the dendritic GluA2 levels. 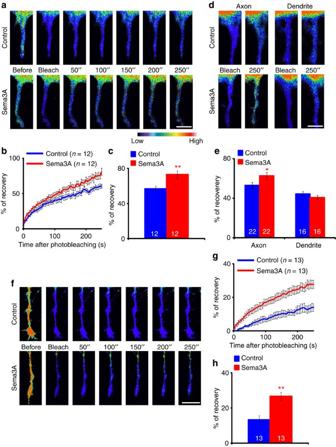Figure 3: Sema3A enhances dendritic transport of GRIP1 and GluA2. (a) Sema3A enhanced fluorescence recovery of the ratio of EGFP-GRIP1 to mcherry within the photobleached area of hippocampal dendrite at 3DIV from 7–11 min after bath application of Sema3A. Average time course and mean fluorescence recovery at 200 s –250 s after photobleaching are shown in (b) and (c), respectively (n=12 neurons from more than three independent cultures). (d) Local application of Sema3A at the axonal growth cone, but not dendritic growth cone, enhanced EGFP-GRIP1 transport along dendrite at 3DIV. Mean fluorescence recovery at 200–250 s after photobleaching is shown ine(n=16–22 neurons from more than three independent cultures). (f) Sema3A enhanced fluorescence recovery of the ratio of EGFP-GluA2 to mcherry within the photobleached area of hippocampal dendrite at 6DIV from 7 to 11 min after bath application of Sema3A. Average time course and mean fluorescence recovery at 200 to 250 s after photobleaching are shown in (g) and (h), respectively (n=13 neurons from three independent cultures). The magnitude of the ratio of fluorescent intensity is expressed by pseudo-colour in a linear scale (a; red and purple representing the highest and lowest, respectively). Scale bars, 5 μm. *P<0.05, **P<0.01 byt-test compared with vehicle control. Data are presented as mean±s.e.m. Figure 3: Sema3A enhances dendritic transport of GRIP1 and GluA2. ( a ) Sema3A enhanced fluorescence recovery of the ratio of EGFP-GRIP1 to mcherry within the photobleached area of hippocampal dendrite at 3DIV from 7–11 min after bath application of Sema3A. Average time course and mean fluorescence recovery at 200 s –250 s after photobleaching are shown in ( b ) and ( c ), respectively ( n =12 neurons from more than three independent cultures). ( d ) Local application of Sema3A at the axonal growth cone, but not dendritic growth cone, enhanced EGFP-GRIP1 transport along dendrite at 3DIV. Mean fluorescence recovery at 200–250 s after photobleaching is shown in e ( n =16–22 neurons from more than three independent cultures). ( f ) Sema3A enhanced fluorescence recovery of the ratio of EGFP-GluA2 to mcherry within the photobleached area of hippocampal dendrite at 6DIV from 7 to 11 min after bath application of Sema3A. Average time course and mean fluorescence recovery at 200 to 250 s after photobleaching are shown in ( g ) and ( h ), respectively ( n =13 neurons from three independent cultures). The magnitude of the ratio of fluorescent intensity is expressed by pseudo-colour in a linear scale ( a ; red and purple representing the highest and lowest, respectively). Scale bars, 5 μm. * P <0.05, ** P <0.01 by t -test compared with vehicle control. Data are presented as mean±s.e.m. Full size image To investigate possible involvement of protein synthesis in dendritic localization of GluA2, we examined the effect of cycloheximide (CHX), a protein synthesis inhibitor, at the concentration of 25 μM which almost completely inhibits protein synthesis in cultured hippocampal neurons [28] . Sema3A enhanced immunostaining of GluA2 in both soma and dendrites. CHX, when applied to somatodendrite region using the microfluidic culture system, suppressed the action of Sema3A on the GluA2 levels in soma (Sema3A: 154.5±14.2%, n =19; Sema3A+CHX: 132.3±15.0%, n =17; Supplementary Fig. 3b,c ). CHX partially suppressed Sema3A-enhanced immunostaining of GluA2 in dendrites (Sema3A: 220.1±12.6%, n =19; Sema3A+CHX: 160.6±13.3%, n =17; Supplementary Fig. 3b,c ). These results suggest that Sema3A also enhances the translation of GluA2 and that both newly generated and pre-existing GluA2 are anterogradely transported along dendrites through GRIP1/KIF5 complex. To examine the possible role of protein degradation, we examined the effects of leupeptin (50 μM) and MG132 (10 μM), inhibitions of lysosomal and proteasomal protein degradation, respectively [29] , [30] . Both the regents did not affect the Sema3A-induced GluA2 localization, suggesting that the action of Sema3A is not due to a change in the rate of protein degradation ( Supplementary Fig. 3d,e ). Dynein motor complex mediates the Sema3A-induced signal The cytoplasmic dynein complex functions as a motor for intracellular retrograde transport [31] . We sought to determine whether retrograde axonal transport is involved in the propagation of Sema3A signal that initiated the dendritic localization of GluA2. Transfection of cytoplasmic dynein heavy chain (cDHC)-siRNA plasmid [32] , which reduced the expression of cDHC ( Supplementary Fig. 4a,e ), attenuated Sema3A-enhanced immunostaining of GluA2 in dendrites (98.7±7.7%, n =67; Fig. 4a,b ). We also examined the effect of dynamitin overexpression in cultured neurons. It is known that dynamitin, a subunit of the dynactin complex, links dynein to cargos. When overexpressed, dynamitin dissociates the dynactin complex in HeLa cell lines [33] . Overexpression of dynamitin selectively suppressed retrograde transport ( Supplementary Fig. 4b ) and attenuated Sema3A-enhanced immunostaining of GluA2 (104.7±7.7%, n =69; Supplementary Fig. 4c,d ). These findings suggest that retrograde transport is involved in Sema3A-induced dendritic localization of GluA2. 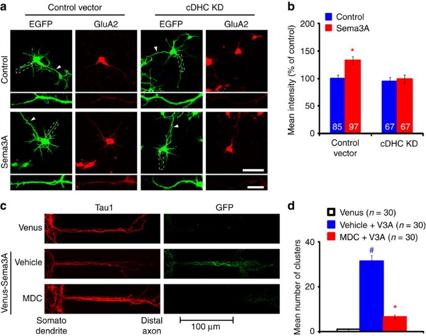Figure 4: The dynein-dependent retrograde transport mediates Sema3A-induced dendritic localization of GluA2. (a) Knockdown of cDHC-attenuated Sema3A-enhanced immunostaining of GluA2 in dendrites. Magnified images of boxed areas in upper panels are shown in lower panels. Arrowheads indicate axon. Normalized mean immunostaining intensity of dendrite per neuron is shown inb(n=67–97 neurons from more than three independent cultures). (c) Venus-Sema3A (V3A) was locally applied at distal axon using the microfluidic culture system. Thirty minutes later, fluorescence signals of Venus-Sema3A (V3A), but not Venus alone, were observed along the axon. The mean number of Venus or Venus-Sema3A clusters observed in proximal axon (within 100 μm from the initiation) is shown ind(n=30 neurons from three independent cultures). Pretreatment with MDC at distal axon suppressed the axonal distribution of Venus-Sema3A. Scale bars, 50 μm (upper panel); 10 μm (lower panel). *P<0.01 by ANOVA compared with vehicle control (b) or vehicle+Sema3A (d).#P<0.01 by ANOVA compared with Venus (d). Data are presented as mean±s.e.m. Figure 4: The dynein-dependent retrograde transport mediates Sema3A-induced dendritic localization of GluA2. ( a ) Knockdown of cDHC-attenuated Sema3A-enhanced immunostaining of GluA2 in dendrites. Magnified images of boxed areas in upper panels are shown in lower panels. Arrowheads indicate axon. Normalized mean immunostaining intensity of dendrite per neuron is shown in b ( n =67–97 neurons from more than three independent cultures). ( c ) Venus-Sema3A (V3A) was locally applied at distal axon using the microfluidic culture system. Thirty minutes later, fluorescence signals of Venus-Sema3A (V3A), but not Venus alone, were observed along the axon. The mean number of Venus or Venus-Sema3A clusters observed in proximal axon (within 100 μm from the initiation) is shown in d ( n =30 neurons from three independent cultures). Pretreatment with MDC at distal axon suppressed the axonal distribution of Venus-Sema3A. Scale bars, 50 μm (upper panel); 10 μm (lower panel). * P <0.01 by ANOVA compared with vehicle control ( b ) or vehicle+Sema3A ( d ). # P <0.01 by ANOVA compared with Venus ( d ). Data are presented as mean±s.e.m. Full size image Sema3A enhances the transport of Sema3A signal components Neurotrophins induce the retrograde axonal transport of their active signal components to transmit survival signals from distal axon to somatodendrite [34] . We hypothesized that Sema3A may induce the retrograde axonal transport of signalling components of both itself and its receptor complex. In an attempt to visualize the localization of Sema3A in an activated distal axon, we locally applied Venus-Sema3A [35] to distal axon using the microfluidic culture system. At 30 min after stimulation, Venus-Sema3A emerged as punctate signals from the distal axon leading up to the somatodendrite, whereas Venus alone did not show any punctate signals along the axon ( Fig. 4c,d ). In addition, local treatment of the distal axon with monodansylcadaverine (MDC) (100 μM), an inhibitor of clathrin-dependent endocytosis, suppressed this axonal distribution of Venus-Sema3A ( Fig. 4c,d ). This is consistent with the previous finding that Sema3A is internalized through a clathrin-dependent mechanism [36] . These results suggest that Sema3A is internalized at distal axon and then retrogradely transported along the axon. PlexA4 was shown to be a signal-transducing component of Sema3A in vivo [37] . The knockdown of PlexA4 ( Supplementary Fig. 5 ) suppressed Sema3A-enhanced immunostaining of GluA2 in dendrites (119.8±4.7%, n =50), which was rescued by expressing a siRNA-resistant form of PlexA4 (147.6±9.0%, n =50; Fig. 5 ). We therefore examined the distribution of PlexA4 with or without Sema3A in cultured hippocampal neurons. Anti-PlexA4 immunostaining signals were mainly observed in distal axons in non-treated neurons. The PlexA4 signals were markedly decreased in the distal axon, but increased in the soma in parallel in neurons treated with Sema3A for 10 min. Some faint anti-PlexA4 staining could be observed in dendrites in 20 min, and clearly observed in 30 min after Sema3A stimulation, respectively ( Fig. 6a,b ). This result suggests that Sema3A induces a retrograde axonal transport and then dendritic transport of PlexA4. To directly monitor the transport of PlexA4, we performed FRAP analysis on the cultured hippocampal neurons expressing PlexA4-EGFP. From 1 to 5 min after Sema3A stimulation, fluorescence recovery of PlexA4-EGFP was accelerated in the photobleached area of axons, while there was no change in that of dendrites ( Fig. 6c,d ). From 13 to 17 min after Sema3A stimulation, however, fluorescence recovery of PlexA4-EGFP in the photobleached area was accelerated in dendrites, while there was no change in axons ( Fig. 6e,f ). This finding indicates that Sema3A first facilitated PlexA4 transport in axons and then in dendrites. 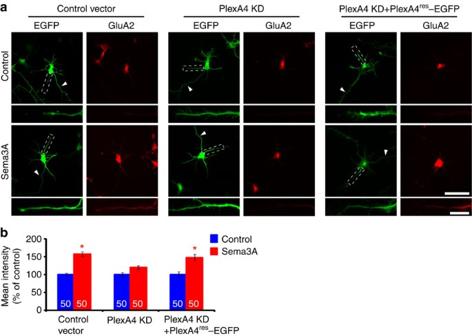Figure 5: PlexA4 mediates Sema3A-induced dendritic localization of GluA2. (a) Knockdown of PlexA4 attenuated Sema3A-enhanced immunostaining of GluA2 in dendrites. This attenuation was rescued by expressing a PlexA4-EGFPres. Magnified images of boxed areas in upper panels are shown in lower panels. Arrowheads indicate axon. Normalized mean immunostaining intensity of dendrite per neuron is shown inb(n=50 neurons from three independent cultures). Scale bars, 50 μm (upper panel); 10 μm (lower panel). *P<0.01 by ANOVA compared with vehicle control. Data are presented as mean±s.e.m. Figure 5: PlexA4 mediates Sema3A-induced dendritic localization of GluA2. ( a ) Knockdown of PlexA4 attenuated Sema3A-enhanced immunostaining of GluA2 in dendrites. This attenuation was rescued by expressing a PlexA4-EGFP res . Magnified images of boxed areas in upper panels are shown in lower panels. Arrowheads indicate axon. Normalized mean immunostaining intensity of dendrite per neuron is shown in b ( n =50 neurons from three independent cultures). Scale bars, 50 μm (upper panel); 10 μm (lower panel). * P <0.01 by ANOVA compared with vehicle control. Data are presented as mean±s.e.m. 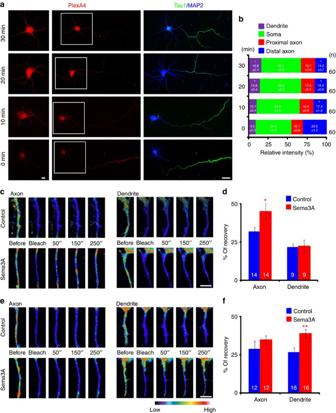Figure 6: Sema3A enhances PlexA4 transport in axons and in dendrites. (a) Sema3A decreased the levels of PlexA4 immunostaining in distal axon and then increased the levels in dendrites. Magnified images of boxed areas in middle panels are shown in left panels. Relative mean immunostaining intensity in distal axon, proximal axon, soma and dendrites per neuron according to the counter staining of Tau1 (axon) and MAP2 (dendrites) is shown inb(n=60 neurons from three independent cultures). (c) Sema3A enhances fluorescence recovery of the ratio of PlexA4-EGFP to mcherry within the photobleached area of hippocampal axon, but not dendrite, from 1 to 5 min after Sema3A stimulation. Mean fluorescence recovery at 200–250 s after photobleaching is shown ind(n=9–14 neurons from more than three independent cultures). (e) Sema3A enhances fluorescence recovery of PlexA4-EGFP in the photobleached area of hippocampal dendrite, but not axon, from 13 to 17 min after Sema3A stimulation. Mean fluorescence recovery at 200–250 s after photobleaching is shown inf(n=12–16 neurons from more than three independent cultures). Scale bars ina, 5 μm (left panel); 20 μm (right panel); (c,e), 5 μm.†P<0.01 by ANOVA compared with 0 min. *P<0.05, **P<0.01 byt-test compared with vehicle control. Data are presented as mean±s.e.m. Full size image Figure 6: Sema3A enhances PlexA4 transport in axons and in dendrites. ( a ) Sema3A decreased the levels of PlexA4 immunostaining in distal axon and then increased the levels in dendrites. Magnified images of boxed areas in middle panels are shown in left panels. Relative mean immunostaining intensity in distal axon, proximal axon, soma and dendrites per neuron according to the counter staining of Tau1 (axon) and MAP2 (dendrites) is shown in b ( n =60 neurons from three independent cultures). ( c ) Sema3A enhances fluorescence recovery of the ratio of PlexA4-EGFP to mcherry within the photobleached area of hippocampal axon, but not dendrite, from 1 to 5 min after Sema3A stimulation. Mean fluorescence recovery at 200–250 s after photobleaching is shown in d ( n =9–14 neurons from more than three independent cultures). ( e ) Sema3A enhances fluorescence recovery of PlexA4-EGFP in the photobleached area of hippocampal dendrite, but not axon, from 13 to 17 min after Sema3A stimulation. Mean fluorescence recovery at 200–250 s after photobleaching is shown in f ( n =12–16 neurons from more than three independent cultures). Scale bars in a , 5 μm (left panel); 20 μm (right panel); ( c , e ), 5 μm. † P <0.01 by ANOVA compared with 0 min. * P <0.05, ** P <0.01 by t -test compared with vehicle control. Data are presented as mean±s.e.m. Full size image To further investigate the localization of the signalling components, PlexA4, NRP1 and Sema3A, we locally applied Venus-Sema3A to distal axons, fixed and then performed triple immunostaining of Venus-Sema3A (green fluorescent protein (GFP) antibody)/NRP1/MAP2 and Venus-Sema3A/PlexA4/MAP2. When Venus-Sema3A was applied at distal axon, the punctuate signals of NRP1 or PlexA4 were double positive with Venus-Sema3A in MAP2-negative axons ( Supplementary Fig. 6a,b ). This result suggests that Sema3A/NRP1/PlexA4 complex is formed in axons and then transported to somatodendrite ( Supplementary Fig. 6c ). A PlexA4–GluA2 interaction for dendritic GluA2 localization It is possible that PlexA4 may interact with GluA2, and then escorting GluA2 to distal dendrites ( Supplementary Fig. 6c ). To address this issue, we performed a co-immunoprecipitation assay. GluA2 was associated with PlexA4 expressed in HEK293T cells ( Fig. 7b ; Supplementary Fig. 7a,b ). Furthermore, the three IPT domains of PlexA4 (PlexA4-IPT; Fig. 7a ) interacted with GluA2 ( Fig. 7b ; Supplementary Fig. 7a,b ). The relative ratio of immunoprecipitated GluA2 to PlexA4-IPT (percent of full-length PlexA4) was 99.4±8.7% ( n =3). To confirm this observation, we investigated whether or not only IPT domain deleted-PlexA4 (PlexA4-ΔIPT) interacts with GluA2. When expressed in HEK293T cells, PlexA4-ΔIPT interacted with GluA2 ( Fig. 7c ; Supplementary Fig. 7c,d ), although this interaction with GluA2 was fairly weak than that of full-length PlexA4 and of PlexA4-IPT. The relative ratio of immunoprecipitated GluA2 to PlexA4-ΔIPT (percent of full-length PlexA4) was 9.3±3.6% ( n =3) ( Fig. 7c ; Supplementary Fig. 7c,d ), indicating that the three IPT domain of PlexA4 is the main interacting region with GluA2 ( Fig. 7a ). In contrast, the IPT domain of PlexA4 did not interact with NRP1 ( Fig. 7d ; Supplementary Fig. 7e,f ). The relative ratio of immunoprecipitated NRP1 to PlexA4-IPT (percent of full-length PlexA4) was 2.3±1.0% ( n =3), suggesting that the PlexA4-GluA2 interacting region does not overlap with that of PlexA4-NRP1 ( Fig. 7a ). Co-immunoprecipitation was also performed using rat brain lysates by anti-PlexA4 mouse monoclonal antibody. The product of co-immunoprecipitation was electrophoressed, and then immunoblotted with anti-PlexA4 rabbit polyclonal antibody and anti-GluA2 mouse monoclonal antibody. GluA2 was also associated with PlexA4 in the brain ( Fig. 7e ; Supplementary Fig. 7g,h ). To investigate whether endogenous PlexA4 interacted with GluA2 in cultured hippocampal neurons, we performed the immunostaining using in situ proximity ligation assay (PLA) technology [38] . In the presence of Sema3A, PlexA4-GluA2 interacting signals were first detected in the cell body ( Fig. 7f,g ). The signal clusters accumulated in the cell body followed by dispersing to dendrites ( Fig. 7f,g ). These Sema3A-induced spatially and temporally dependent changes of PlexA4-GluA2 interacting signals corresponded well with those of PlexA4 immunostaining signals ( Fig. 6a,b ). 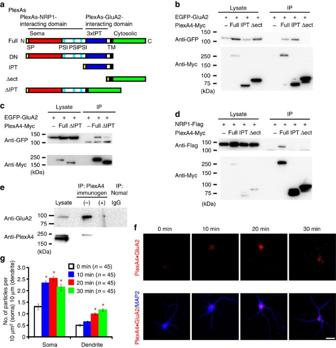Figure 7: PlexA4 interacts with GluA2 through its IPT domain. (a) Structure of PlexAs and schematic representation of constructed PlexAs mutant. PlexAs contain signal peptides, sema domain, three PSI (domains found in plexin, semaphorin and integrin) domains, three IPT (immunoglobulin-like plexin transcription factor) domains, transmembrane domain and cytosolic domain. Abbreviations are as follows: Full, full length; DN, dominant negative; IPT, three IPT; Δect, lacking the entire ectodomain; ΔIPT, lacking three IPT ectodomain. (b) EGFP-tagged GluA2 interacted with full-length or IPT domain of PlexA4-Myc. (c) EGFP-tagged GluA2 weakly interacted with ΔIPT mutant of PlexA4-Myc. (d) Flag-tagged NRP1 interacted with full length, but not IPT domain, of PlexA4-Myc. (e) GluA2 and PlexA4 were co-immunoprecipitated from rat brain lysates. (f) A Sema3A-induced increase in the number of PlexA4–GluA2 interacting signals detected byin situPLA technology in cell body followed by an increase in dendrites. The mean number of PlexA4-GluA2 interacting signals per 10 μm2(soma) or 10 μm (dendrite) is shown ing(n=45 neurons from three independent cultures). Scale bar, 20 μm. *P<0.01 by ANOVA compared with 0 min. Data are presented as mean±s.e.m. Full scan of western blot ofb–eare shown inSupplementary Fig. 7a–g. Figure 7: PlexA4 interacts with GluA2 through its IPT domain. ( a ) Structure of PlexAs and schematic representation of constructed PlexAs mutant. PlexAs contain signal peptides, sema domain, three PSI (domains found in plexin, semaphorin and integrin) domains, three IPT (immunoglobulin-like plexin transcription factor) domains, transmembrane domain and cytosolic domain. Abbreviations are as follows: Full, full length; DN, dominant negative; IPT, three IPT; Δect, lacking the entire ectodomain; ΔIPT, lacking three IPT ectodomain. ( b ) EGFP-tagged GluA2 interacted with full-length or IPT domain of PlexA4-Myc. ( c ) EGFP-tagged GluA2 weakly interacted with ΔIPT mutant of PlexA4-Myc. ( d ) Flag-tagged NRP1 interacted with full length, but not IPT domain, of PlexA4-Myc. ( e ) GluA2 and PlexA4 were co-immunoprecipitated from rat brain lysates. ( f ) A Sema3A-induced increase in the number of PlexA4–GluA2 interacting signals detected by in situ PLA technology in cell body followed by an increase in dendrites. The mean number of PlexA4-GluA2 interacting signals per 10 μm 2 (soma) or 10 μm (dendrite) is shown in g ( n =45 neurons from three independent cultures). Scale bar, 20 μm. * P <0.01 by ANOVA compared with 0 min. Data are presented as mean±s.e.m. Full scan of western blot of b – e are shown in Supplementary Fig. 7a–g . Full size image We next attempted to compare the effect of PlexA4 mutants on GluA2 and PlexA4 immunostaining signals in dendrites. Containing the entire region of PlexA4 ectodomain ( Fig. 7a ), the PlexA4-DN can be recognized by the anti-PlexA4 antibody [39] . To avoid this cross-reaction, we first employed mutant forms of PlexA1, another PlexA family molecule: PlexA1-DN and IPT domain of PlexA1 (PlexA1-IPT). PlexA1-DN was previously shown to inhibit Sema3A-induced signalling [8] . We confirmed that overexpression of PlexA1-DN attenuated the Sema3A-induced increase in the immunostaining of both GluA2 (96.1±12.2%, n =33) and PlexA4 (100.5±5.6%, n =46; Fig. 8a ; Supplementary Fig. 8c,d ). We also generated PlexA1-IPT, which interacted with GluA2, but not NRP1 ( Supplementary Fig. 8a,b,i,j ). Overexpression of PlexA1-IPT suppressed the Sema3A-induced increase in the immunostaining intensity of GluA2 (97.3±8.0%, n =42), while having no effect on the intensity of PlexA4 (126.2±5.9%, n =45; Fig. 8a ; Supplementary Fig. 8c,d ). In addition, overexpression of PlexA1-IPT indeed suppressed the number of PlexA4-GluA2 interacting signals in cultured hippocampal neurons both in soma and dendrites ( Fig. 8b,c ). We confirmed that PlexA4-IPT similarly suppressed the Sema3A-induced immunostaining of GluA2 (99.9±6.2%, n =30; Supplementary Fig. 8e,f ). In contrast to PlexA1-IPT, the knockdown of GRIP1 selectively suppressed the Sema3A-enhanced PlexA4-GluA2 interaction in dendrites but not soma ( Fig. 8d,e ). These results together suggest that PlexA4 interacts with GluA2 through its IPT domain and then escorts GluA2 to dendrites by GRIP1-dependent dendritic transport. This idea is consistent with our finding that, after Sema3A stimulation, PlexA4–GluA2 interaction was first detected in the cell body and thereafter in dendrites ( Fig. 7f,g ). 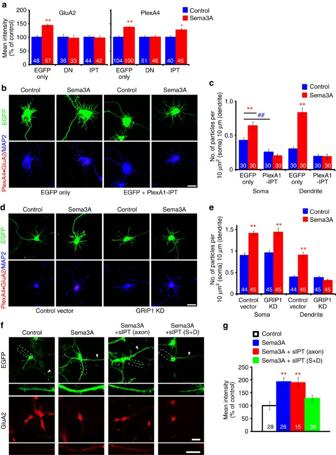Figure 8: GluA2–PlexA interaction in the somatodendritic region is required for Sema3A-induced dendritic localization of GluA2. (a) Overexpression of PlexA1-DN (A1-DN) attenuated Sema3A-enhanced immunostaining of both GluA2 and PlexA4 in dendrites. Overexpression of PlexA1 IPT domain (A1-IPT) attenuated Sema3A-enhanced immunostaining of GluA2 without modifying that of PlexA4 (n=33–104 neurons from more than three independent cultures). To discriminate between endogenous PlexA4 and exogenous PlexA mutants, we utilized mutant forms of PlexA1 instead of PlexA4 that is recognized by the anti-PlexA4 antibody (see text). (b) Overexpression of A1-IPT suppressed the number of PlexA4–GluA2 interaction signals in the soma of the neurons without Sema3A. The A1-IPT also suppressed the number of signals in the soma and dendrites treated with Sema3A for 30 min. The mean number of PlexA4–GluA2 interacting signals per 10 μm2(soma) or 10 μm (dendrite) is shown inc(n=30 neurons from three independent cultures). (d) Knockdown of GRIP1 suppressed Sema3A-induced increase in the number of PlexA4-GluA2 interacting signals in the dendrites but not soma. The mean number of PlexA4–GluA2 interacting signals per 10 μm2(soma) or 10 μm (dendrite) is shown ine(n=44–45 neurons from three independent cultures). (f) Pretreatment with sPlexA1-IPT, using the microfluidic culture system, in the somatodendritic region, but not the axonal region, attenuated the enhanced immunostaining of GluA2 by Sema3A stimulation in the axonal region. Magnified images of boxed areas in upper panels are shown in lower panels. Arrowheads indicate axon. Normalized mean immunostaining intensity of dendrite per neuron is shown ing(n=15–38 neurons from more than three independent cultures). Scale bars inb, d, 20 μm;f, 20 μm (upper panel); 10 μm (lower panel). The representative images ofaare shown inSupplementary Fig. 8c,d. *P<0.05, **P<0.01 by ANOVA compared with vehicle control.##P<0.01 by ANOVA compared with EGFP only. Data are presented as mean±s.e.m. Figure 8: GluA2–PlexA interaction in the somatodendritic region is required for Sema3A-induced dendritic localization of GluA2. ( a ) Overexpression of PlexA1-DN (A1-DN) attenuated Sema3A-enhanced immunostaining of both GluA2 and PlexA4 in dendrites. Overexpression of PlexA1 IPT domain (A1-IPT) attenuated Sema3A-enhanced immunostaining of GluA2 without modifying that of PlexA4 ( n =33–104 neurons from more than three independent cultures). To discriminate between endogenous PlexA4 and exogenous PlexA mutants, we utilized mutant forms of PlexA1 instead of PlexA4 that is recognized by the anti-PlexA4 antibody (see text). ( b ) Overexpression of A1-IPT suppressed the number of PlexA4–GluA2 interaction signals in the soma of the neurons without Sema3A. The A1-IPT also suppressed the number of signals in the soma and dendrites treated with Sema3A for 30 min. The mean number of PlexA4–GluA2 interacting signals per 10 μm 2 (soma) or 10 μm (dendrite) is shown in c ( n =30 neurons from three independent cultures). ( d ) Knockdown of GRIP1 suppressed Sema3A-induced increase in the number of PlexA4-GluA2 interacting signals in the dendrites but not soma. The mean number of PlexA4–GluA2 interacting signals per 10 μm 2 (soma) or 10 μm (dendrite) is shown in e ( n =44–45 neurons from three independent cultures). ( f ) Pretreatment with sPlexA1-IPT, using the microfluidic culture system, in the somatodendritic region, but not the axonal region, attenuated the enhanced immunostaining of GluA2 by Sema3A stimulation in the axonal region. Magnified images of boxed areas in upper panels are shown in lower panels. Arrowheads indicate axon. Normalized mean immunostaining intensity of dendrite per neuron is shown in g ( n =15–38 neurons from more than three independent cultures). Scale bars in b, d , 20 μm; f , 20 μm (upper panel); 10 μm (lower panel). The representative images of a are shown in Supplementary Fig. 8c,d . * P <0.05, ** P <0.01 by ANOVA compared with vehicle control. ## P <0.01 by ANOVA compared with EGFP only. Data are presented as mean±s.e.m. Full size image The suppressive effect of the extracellular IPT domain of PlexA1 on the Sema3A-induced GluA2 localization suggests that PlexA may be a cis-interacting partner of GluA2 at the IPT domain. Because clathrin- and dynamin-mediated endocytosis of GluA2 mainly occurs at the somatodendritic plasma membrane [40] , the Sema3A-induced PlexA–GluA2 interaction may occur in the somatodendritic area. To address this issue, we locally applied the soluble form of alkaline phosphatase (AP)-tagged PlexA1-IPT (sPlexA1-IPT) to a given neuronal compartment by using the microfluidic chamber. When applied locally to the somatodendritic field, sPlexA1-IPT (50 nM) attenuated the Sema3A-enhanced immunostaining of GluA2 in dendrites. In contrast, sPlexA1-IPT applied to the axonal region did not affect the Sema3A action (Sema3A: 192.8±15.6%, n =26; Sema3A+ sPlexA1-IPT at axon: 188.9±20.5%, n =15; Sema3A+ sPlexA1-IPT at somatodendrite: 128.8±12.7%, n =38; Fig. 8f,g ). We further found that sPlexA1-IPT did not affect Sema3A-induced growth cone collapse in cultured hippocampal neurons ( Supplementary Fig. 8g,h ), again indicating that sPlexA1-IPT did not interrupt the ligand–receptor interaction for Sema3A signalling (see above). These data suggest that the GluA2–PlexA interaction in the somatodendritic region is required for the Sema3A effect on dendritic localization of GluA2. Sema3A regulates dendritic patterning via GluA2 localization To address in vivo relevance of the Sema3A function, we compared the distribution of GluA2 and GRIP1 in wild-type ( wt ) and sema3A -deficient mice. In the hippocampus of P0 wt mice, GluA2 and GRIP1 were evenly distributed in stratum lacunosum-moleculare (slm), stratum pyramidale (sp) and stratum radiatum (sr). However, in sema3A -deficient mice, GluA2 and GRIP1 were retained in sp and sr, the layers containing cell bodies and proximal dendrites of pyramidal neurons, respectively ( Supplementary Fig. 9b,c ). In contrast, such a change in localization was not observed for GluA1 ( Supplementary Fig. 9a,c ). These biased GluA2/GRIP1 immunostaining signals towards the proximal dendrites indicate that localization of the GluA2/GRIP1 complex to distal dendrites was impaired in sema3A -deficient mice. We investigated whether the PlexA4–GluA2 interaction is required for the dendritic localization of GluA2 in vivo . To monitor GluA1 and GluA2 localization, we weakly overexpressed HA-tagged GluA1 or GluA2 in the rat CA1 hippocampus at E17 by in utero electroporation. The distribution of HA-GluA1 or -GluA2 was observed at postnatal day 2 (P2) ( Fig. 9a ). When co-expressed with PlexA1-IPT, HA-GluA2 was accumulated at apical side of the perinuclear region of the cell body, whereas HA-GluA2 was distributed up to the apical dendrite without co-expression of PlexA1-IPT ( Fig. 9b–d ). Such altered distribution was not observed with HA-GluA1 ( Fig. 9b–d ). These results indicate that distribution of GluA2 but not GluA1 in dendrites is suppressed by the overexpression of PlexA1-IPT in vivo . These findings suggest that PlexA4–GluA2 interaction is required for Sema3A signalling to drive GluA2 to dendrites in vivo . 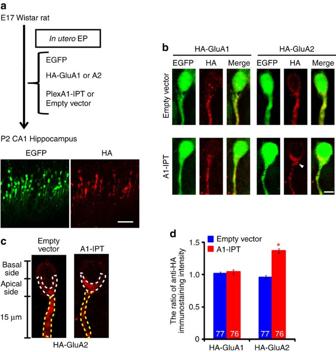Figure 9: The overexpression of PlexA1-IPT suppresses dendritic localization of GluA2in vivo. (a) The scheme of this experiment. EGFP, HA-tagged GluA1 or GluA2 with or without PlexA1-IPT expressing vectors were electroporated into rat CA1 hippocampus at E17, and distribution of HA-GluAs was examined at P2. (b) HA-GluA2 signal, but not GluA1 signal, was retained in the apical side of the perinuclear region of the cell body by overexpression of PlexA1-IPT (arrowhead). (c) HA signals in the apical side of the perinuclear region and proximal apical dendrite region (within 15 μm of the initiation point) are outlined by white and yellow broken lines, respectively. The mean ratios of HA intensities between perinuclear and dendrite regions are shown ind(n=76–77 neurons from three individual brains). Scale bars ina, 50 μm;b, 5 μm. *P<0.01 byt-test compared with without PlexA1-IPT (empty vector). Data are presented as mean±s.e.m. Figure 9: The overexpression of PlexA1-IPT suppresses dendritic localization of GluA2 in vivo . ( a ) The scheme of this experiment. EGFP, HA-tagged GluA1 or GluA2 with or without PlexA1-IPT expressing vectors were electroporated into rat CA1 hippocampus at E17, and distribution of HA-GluAs was examined at P2. ( b ) HA-GluA2 signal, but not GluA1 signal, was retained in the apical side of the perinuclear region of the cell body by overexpression of PlexA1-IPT (arrowhead). ( c ) HA signals in the apical side of the perinuclear region and proximal apical dendrite region (within 15 μm of the initiation point) are outlined by white and yellow broken lines, respectively. The mean ratios of HA intensities between perinuclear and dendrite regions are shown in d ( n =76–77 neurons from three individual brains). Scale bars in a , 50 μm; b , 5 μm. * P <0.01 by t -test compared with without PlexA1-IPT (empty vector). Data are presented as mean±s.e.m. Full size image Sema3A plays an important role in dendritic growth and branching [13] , [14] , [16] , [17] , [41] . To further investigate the functional role of GluA2 localization, we performed knockdown of GluA2 and examined the effect of Sema3A on dendritic branching in cultured hippocampal neurons. The neurons at 6DIV were stimulated with Sema3A for 24 h (7DIV), and fixed for immunostaining. The knockdown of GluA2 attenuated Sema3A-induced dendritic branching, and this effect was rescued by expressing a siRNA-resistant form of GluA2 ( Fig. 10a,b ; Supplementary Fig. 10 ). We next overexpressed PlexA1-IPT by in utero electroporation at E17, and investigated the dendritic morphology at P15. In the absence of PlexA1-IPT, the first branch was mainly observed near the slm region ( Fig. 10c,d ). In PlexA1-IPT overexpressed neurons, the apical dendrites branched shortly after they enter the sr region, showing proximal bifurcation, a similar phenotype to that seen in sema3A -deficient mice [14] , [17] . This result suggests that the PlexA4–GluA2 interaction is required for Sema3A to regulate dendritic patterning through the localization of GluA2 both in vitro and in vivo . 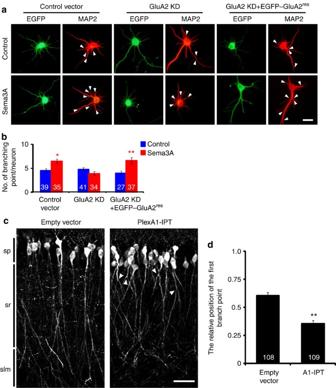Figure 10: The Sema3A-enhanced dendritic GluA2 regulates dendritic patterning bothin vitroandin vivo. (a) Knockdown of GluA2-suppressed Sema3A-induced dendritic branching of cultured hippocampal neurons. This knockdown effect was rescued by expressing a EGFP-GluA2res. Arrowheads indicate MAP2-positive dendritic branching point. Normalized mean number of dendritic branching points per neuron is shown inb(n=27–41 neurons from more than three independent cultures). (c) Compared with empty-vector-electroporated neurons, apical dendrites branched shortly after they enter the sr region in the PlexA1-IPT overexpressed neurons (arrowheads). The relative position of the first branch point of apical dendrite is shown ind(n=108–109 neurons from three individual brains). The relative length of the sr was set to 1 (position 0 is the border between sp and sr, position 1 the border between sr and slm). Scale bars ina, 25 μm;c, 50 μm. *P<0.05, **P<0.01 by ANOVA compared with vehicle control (b) ort-test compared with without PlexA1-IPT (empty vector,d). sp, stratum pyramidale; sr, stratum radiatum; slm, stratum lacunosum-moleculare. Data are presented as mean±s.e.m. Figure 10: The Sema3A-enhanced dendritic GluA2 regulates dendritic patterning both in vitro and in vivo . ( a ) Knockdown of GluA2-suppressed Sema3A-induced dendritic branching of cultured hippocampal neurons. This knockdown effect was rescued by expressing a EGFP-GluA2 res . Arrowheads indicate MAP2-positive dendritic branching point. Normalized mean number of dendritic branching points per neuron is shown in b ( n =27–41 neurons from more than three independent cultures). ( c ) Compared with empty-vector-electroporated neurons, apical dendrites branched shortly after they enter the sr region in the PlexA1-IPT overexpressed neurons (arrowheads). The relative position of the first branch point of apical dendrite is shown in d ( n =108–109 neurons from three individual brains). The relative length of the sr was set to 1 (position 0 is the border between sp and sr, position 1 the border between sr and slm). Scale bars in a , 25 μm; c , 50 μm. * P <0.05, ** P <0.01 by ANOVA compared with vehicle control ( b ) or t -test compared with without PlexA1-IPT (empty vector, d ). sp, stratum pyramidale; sr, stratum radiatum; slm, stratum lacunosum-moleculare. Data are presented as mean±s.e.m. Full size image Numerous cell adhesion molecules and extracellular matrix proteins participate in branching or synapse formation by locally affecting the site of axodendritic contacts [42] . In addition to this local event, it was previously reported that development of the dendrites of some neurons is delayed until their axons have reached their targets [43] . This observation suggested that a retrograde signal transmitted from the axon terminals to the cell body is required for the initiation of dendrite development. Our study revealed that, in hippocampal neurons at an early developmental stage, PlexA4 mediates retrograde Sema3A signalling from the axonal growth cone, acts as a cis-interacting receptor with GluA2 in somatodendritic regions, and escorts GluA2 to the distal dendrites ( Supplementary Fig. 6c ). Our model proposes a novel form of regulation of AMPA receptor localization by retrograde axonal transport, highlighting diverse physiological roles of axon guidance molecules. Target-derived neurotrophins activate tropomyosin-related kinase receptors (Trks) and are endocytosed by clathrin-dependent and -independent mechanisms into signalling endosomes. This signal is transmitted from axonal growth cones to cell bodies or dendrites to direct neurite growth, survival and cell migration via dynein-dependent transport [44] . When applied at the axonal growth cone, Sema3A facilitates dendritic transport ( Supplementary Fig. 1c ). Consistent with this finding, the site of Sema3A action was restricted at the axonal growth cone to regulate the dendritic localization of GluA2 and GRIP1 ( Figs 1b,c and 3d,e ). These results indicate that the Sema3A-induced signal at the axonal growth cone is propagated by some mechanisms to axon and somatodendrite. Knockdown of cDHC suppressed the Sema3A-induced increase in the GluA2 immunostaining signal ( Fig. 4a,b ). In addition, Venus-Sema3A applied at the distal axons was retrogradely transported along the axon ( Fig. 4c,d ). Sema3A first decreased PlexA4 levels in the distal axon, and then increased PlexA4 levels in the soma thereafter in the dendrites. This distributional change was associated with acceleration of axonal and dendritic transport of PlexA4-EGFP ( Fig. 6 ). Thus, Sema3A induces dynein-dependent retrograde axonal transport of its active signal components, suggesting that the Sema3A-induced signal is transmitted by signalling endosomes. However, several differences may exist between Sema3A and neurotrophins. For example, neurotrophins play roles in dendritic growth and synapse formation through a cascade of phosphorylation events through Trks [45] . To date, no direct interaction between Trks and AMPA receptor subunits has been proven. We found that the interaction between PlexA4 and GluA2 was essential for GluA2 delivery to dendrites. PlexA4 and GluA2 were co-immunoprecipitated from rat brain lysates ( Fig. 7e ). The PlexA4–GluA2 interacting signals were first observed in the cell body and then localized to dendrites by GRIP1-dependent dendritic transport ( Figs 7f,g and 8d,e ). GluA2 mainly interacted with the IPT domain of PlexA1 and PlexA4 ( Fig. 7b,c ; Supplementary Fig. 8a,b,i,j ). Overexpression of PlexA1-IPT suppressed PlexA4–GluA2 interaction ( Fig. 8b,c ) and Sema3A-induced increase in the immunostaining intensity of GluA2; however, it did not modify the Sema3A-induced increase in PlexA4 levels in dendrites ( Fig. 8a ; Supplementary Fig. 8c,d ). In contrast, overexpression of PlexA1-DN suppressed the Sema3A-induced increase in the intensities of both GluA2 and PlexA4 ( Fig. 8a ; Supplementary Fig. 8c,d ). Hence, the attenuated Sema3A-induced increase in GluA2 intensity is probably due to the disruption of the PlexA4–GluA2 interaction at IPT, but not impairment of Sema3A signalling per se . These findings indicate that the interaction between GluA2 and PlexA4 is essential for dendritic GluA2 localization. Because the effect of Sema3A on dendritic GluA2 localization was attenuated by somatodendritic application but not axonal application of sPlexA1-IPT ( Fig. 8f,g ), PlexA4 may interact with GluA2 mainly in the cell body. Consistently, the PlexA4–GluA2 interaction signals were first detected in the cell body followed by detection in dendrites ( Fig. 7f,g ). Because sPlexA1-IPT applied extracellularly to somatodendritic regions suppressed the Sema3A effect, PlexA might interact with GluA2 at the outer surface of cell bodies. On the other hand, inhibition of protein synthesis at somatodendrite region partially suppressed Sema3A-induced immunostaining of GluA2 in dendrites ( Supplementary Fig. 3b,c ), suggesting that Sema3A also enhances the translation of GluA2. This finding suggests that both newly generated and pre-existing GluA2 are anterogradely transported along dendrites. AMPA receptors are assembled in the endoplasmic reticulum and Golgi apparatus in the soma and dendrites and are delivered into the dendrite via kinesin-dependent vesicular trafficking. Mature AMPA receptors undergo constitutive recycling through endosomal trafficking pathway [46] . Therefore, it is also possible that sPlexA1-IPT is endocytosed upon Sema3A stimulation and thereafter suppresses the endogenous PlexA–GluA2 interaction on the inner surface of the endoplasmic reticulum, Golgi apparatus and signalling endosomes. Further studies are required to delineate how and where the PlexA–GluA2 interaction occurs in cell surface membrane and/or subcellular compartments in neurons. Consistent with the phenotype observed in sema3A -deficient mice ( Supplementary Fig. 9 ), a defect in GluA2 localization in apical dendrites was also seen in PlexA1-IPT-expressing neurons ( Fig. 9 ). We further found that the knockdown of GluA2 attenuated Sema3A-induced dendritic branching in vitro and that overexpression of PlexA-IPT caused proximal bifurcation phenotype in vivo ( Fig. 10 ). Thus, the interaction between GluA2 and PlexA4 is essential for Sema3A to regulate dendritic patterning. GluA2 has been shown to play an important role in dendritic development [47] . GluA2, but not GluA1, regulates dendritic development by recruiting N-cadherin through direct interaction [48] . Drosophila N-cadherin is essential for proper dendritic refinement [49] . Hence it is likely that a decrease in the density of GluA2 in distal dendrites may result in weakening of N-cadherin-regulated dendritic development causing a bifurcation phenotype. Taken together, our findings show that Sema3A plays a role in regulating dendritic development of the hippocampal pyramidal neurons through the regulation of dendritic localization of GluA2. In conclusion, we propose a model in which Sema3A acting on the distal axon regulates GluA2 localization and dendritic development through dynein- and PlexA4-dependent retrograde signalling. In addition to serving as a Sema3A signal-transducing receptor, PlexA may function as a novel regulator of AMPA receptor localization. Cell culture and recombinant protein Hippocampal neurons from male and female Wistar rat at E18 (Charles River Laboratories) were cultured on 0.01% poly- L -lysine (Wako Pure Chemicals) coated dish in neurobasal medium (Invitrogen) supplemented with 2% B27 supplement (Invitrogen) and 0.5 mM L -glutamine (Sigma). The hippocampal neurons were cultured for 3 days unless otherwise noted. Recombinant Sema3A, Venus-Sema3A [35] and soluble form of AP-PlexA1-IPT were prepared using TALON Metal Affinity Resin (Takara) through their histidine tag [10] . To estimate the activity of Sema3A and Venus-Sema3A, DRG from chick at E7 were explanted onto 0.01% poly- L -lysin and 8 μg ml −1 of laminin-coated dish in Ham’s F-12 medium (Wako Pure Chemicals) supplemented with 10% FBS and 10 ng ml −1 NGF (Wako Pure Chemicals). One day later, explants were incubated with Sema3A or Venus-Sema3A, for 30 min at 37 °C followed by fixation and staining with Alexa488-phalloidin (Invitrogen). The percentage of collapsed growth cones was then counted. The concentration that induces 50% of growth cone collapse was set to 0.1 nM [10] . The concentration of AP-tagged proteins was determined based on their AP activity. All animals were handled according to the guidelines outlined in the Institutional Animal Care and Use Committee of the Yokohama City University School of Medicine. Immunocytochemistry Immunocytochemistry was done by a standard protocol under permeabilization with 0.1% TritonX-100 (ref. 50 ). The antibodies used for staining the cultured neurons were as follows: anti-GluA1 rabbit polyclonal antibody (1:500 dilution, provided by K. Kameyama), anti-GluN1 mouse monoclonal antibody (556308, 1:100 dilution, BD Biosciences), anti-GluA2 mouse monoclonal antibody (MAB397, 1:500 dilution, Millipore), anti-GluA3 rabbit polyclonal antibody (GluR3C-Rb-Af1090, 1:200 dilution, Frontier Institute), anti-GRIP1 mouse monoclonal antibody (611319, 1:1,000 dilution, BD Biosciences), anti-Tau1 mouse monoclonal antibody (MAB3420, 1:500 dilution, Millipore), anti-MAP2 rabbit polyclonal antibody (PRB-547C, 1:500 dilution, Covance), anti-MAP2 mouse monoclonal antibody (M1406, 1:1,000 dilution, Sigma), anti-GFP rabbit polyclonal antibody (598, 1:1,000 dilution, MBL), anti-PlexA4 hamster monoclonal antibody [39] (1:500 dilution) and anti-NRP1 rabbit polyclonal antibody (1:1,000 dilution, provided by T. Kawasaki). To investigate the PlexA4 and GluA2 interaction in cultured hippocampal neurons, we performed double immunostaining of anti-PlexA4 hamster monoclonal and anti-GluA2 mouse monoclonal antibodies. The neurons were counter-stained by anti-MAP2 rabbit polyclonal antibody, and the PlexA4–GluA2 interacting signals were visualized by Duolink in situ PLA kits (OLINK Bioscience) according to the manufacturer’s instructions. Immunostained neurons were analysed using a laser scanning microscope (LSM510) with a water-immersed objective lens at × 40 (C-Apochromat/1.2W corr) equipped with an Axioplan 2 imaging microscope (Carl Zeiss). To visualize the surface expression level of GluA2, we performed immunocytochemistry with anti-GluA2 mouse monoclonal antibody (1:50 dilution) under non-permeabilization condition. Cultured neurons are then permeabilized with 0.1% TritonX-100 and counterstained by anti-MAP2 rabbit polyclonal antibody. Immunostained neurons were analysed using a laser scanning microscope (LSM700) with a water-immersed objective lens at × 40 (C-Apochromat/1.2W Korr M27) equipped with an AxioImager Z1 imaging microscope (Carl Zeiss). Immunostaining intensity measurement ImageJ software was used to measure the mean immunostaining intensities stained by anti-GluN1, -GluA1, -GluA2, -GluA3, -GRIP1 or -PlexA4 antibodies. The cultured neurons were treated with Sema3A for 30 min and then fixed for staining. To obtain the mean intensity of dendrite per neuron, immunostaining intensity of each MAP2 or EGFP-positive dendrites was normalized by the volume of dendrites. In EGFP expressing neurons, the longest neurite was defined as axon (indicated by arrowheads in figures). Intensity measurement was performed blindly. To quantify the distributional change of PlexA4 ( Fig. 6a ), the mean intensity of PlexA4 in distal axon (within 20 μm of the axon tip), proximal axon (within 20 μm of the initiation point), soma and dendrites were measured according to the morphology visualized by anti-Tau1 and anti-MAP2 immunocytochemistry. The relative immunostaining intensity of each area of these four regions was calculated. Cell culture in microfluidic chamber Dissociated hippocampal neurons were first transfected with EGFP expression vector using Amaxa rat neuron nucleofector kit (Lonza), according to the manufacturer’s instructions. Neurons were then plated onto one of the reservoirs of AXIS (AX150, Millipore) and cultured for 3 days. For local stimulation by Sema3A (5 nM), each reservoir for axonal or somatodendritic compartment was maintained fluidically isolated by using a small hydrostatic pressure [23] . The EGFP-positive neurons extending long neurites into the axonal regions were used for the analysis ( Supplementary Fig. 1d,e ). To examine the distribution of Venus-Sema3A, dissociated hippocampal neurons were cultured in microfluidic chamber. The purified Venus protein (5 nM) or Venus-Sema3A (5 nM) was then locally applied in the axonal region after 3 days in culture. Thirty minutes later, immunostaining of anti-GFP chicken polyclonal antibody (GFP-1010, 1:5,000 dilution, AVES) with anti-Tau1 monoclonal antibody, anti-NRP1 rabbit polyclonal and anti-MAP2 mouse monoclonal antibodies or anti-PlexA4 hamster monoclonal and anti-MAP2 mouse monoclonal antibodies was performed. MDC (100 μM), when used, was applied in the axonal region 7 min before the application of Venus-Sema3A. To quantify the Venus fluorescent signals, the mean number of Venus only or Venus-Sema3A clusters in the proximal axon within 100 μm from the initiation point were counted. siRNA For knockdown of GRIP1, cDHC, GluA2 or PlexA4, we used siRNA based on pSilencer 3.0 (Ambion). The target sequences were as follows: GRIP1 (ref. 26 ): 5′-GCCAAGAGTGTCCAACCTG-3′, cDHC [32] : 5′-GGGAGGAGGTTATGTTTAA-3′, 5′-GGTGACAGCTTTCGAATGA-3′, 5′-CCAAATACCTACATTACTT-3′ and 5′-GCTCAAACATGACAGAATT-3′, GluA2 (ref. 47 ): 5′-GGAGCACTCCTTAGCTTGA-3′, PlexA4: 5′-GAGCAAGCTAGAGTATGCCACTGAT-3′. A sequence that did not share sequence homology with any rat mRNAs (5′-CAGTCGCGTTTGCGACTGG-3′) was used as the negative control (control vector). The efficacy of siRNA expressing plasmids transfected by Amaxa rat neuron nucleofector kit with a EGFP expressing plasmid into cultured neurons was evaluated by immunoblot analysis of anti-GRIP1 mouse monoclonal (1:2,500 dilution), anti-dynein HC rabbit polyclonal (sc-9115, 1:1,000 dilution, Santa Cruz Biotechnology), anti-PlexA4 rabbit polyclonal (ab39350, 1:2,500 dilution, Abcam), anti-GluA2 mouse monoclonal (1:1,000 dilution), anti-GFP mouse monoclonal (sc-9996, 1:2,500 dilution, Santa Cruz Biotechnology) or anti-β-actin mouse monoclonal (A5316, 1:10,000 dilution, Sigma) antibodies ( Supplementary Figs 2, 4, 5 and 10 ). For the rescue experiment of siRNA of GRIP1, GluA2 and PlexA4, we generated following mutants without changing the amino-acid sequence; rat GRIP1 mRNA (NM_032069) corresponding to nucleotides 417–435 was replaced with GCCTCGAGTTAGTAATCTG; rat GluA2 mRNA (NM_032069) corresponding to nucleotides 829–848 was replaced with GGTGCTTTACTAAGCTTAA; mouse PlexA4 mRNA (NM_175750) corresponding to nucleotides 5,156–5,180 was replaced with GAGCAAACTCGAGTACGCTACTGAC. These mutants tagged with EGFP were co-transfected with siRNA vector. To assess Sema3A-enhanced immunostaining of GluA2, neurons were co-transfected with siRNA plasmid together with EGFP or EGFP-tagged siRNA-resistant mutants expressing vectors by Amaxa rat neuron nucleofector kit. On 3DIV, immunocytochemistry was performed after stimulation with Sema3A for 30 min. To examine the Sema3A-induced dendritic branching, neurons were co-transfected with siRNA expression vector together with EGFP or siRNA-resistant form of GluA2 expressing vector on 3DIV by lipofectoamine2000 transfection regent (Invitrogen). On 6DIV, bath application of Sema3A (5 nM) was performed. After incubation with Sema3A for 24 h, neurons were fixed for immunostaining with anti-GFP chicken polyclonal and anti-MAP2 mouse monoclonal antibodies. The number of MAP2-positive dendritic branch points of EGFP-positive neurons was then counted. Time-lapse observation Using a calcium phosphate method, the neurons were transfected with expression plasmid encoding EGFP-GRIP1 or PlexA4-EGFP on 1DIV or EGFP-GluA2 on 3DIV. We also expressed mcherry to perform ratiometric imaging because it was not photobleached by a 488-nm laser. On 3DIV (EGFP-GRIP1 or PlexA4-EGFP) or 6DIV (EGFP-GluA2), bath application of Sema3A or local application to axonal or dendritic growth cone of Sema3A was performed. After incubation with Sema3A for a desired time frame, a distal dendrite (within 10 μm from the dendrite tip) or the proximal part of axon 15–25 μm away from the cell body in mcherry and EGFP double positive neurons was photobleached with 200 laser irradiations (488 nm) and then imaged at 5-s intervals using a LSM5 PASCAL with an oil-immersed objective lens at 63 × (C-Apochromat/1.4F corr) equipped with an Axioplan 2 imaging microscope (Carl Zeiss). Fluorescence intensity of the ratio of EGFP-fused proteins to mcherry within the outline of the photobleached area was measured by using LSM 5 Image software. Because nonpalmitoylated GRIP1 is associated with intracellular GluA2 (ref. 51 ), we used GRIP1a, a non-palmitoylated splicing isoform [52] , expressing vector throughout the experiments. Immunoprecipitation E18 rat brain samples were homogenized in immunoprecipitation buffer (20 mM Tris-HCl (pH 8.0), 100 mM NaCl, 10 mM NaF, 1 mM Na 3 VO 4 , 1 mM EDTA, 1% Nonidet P-40, cOmplete Mini protease inhibitor cocktail (Roche)). The lysates were centrifuged at 15,000 r.p.m. for 20 min at 4 °C. The supernatant were then incubated with 1 μg of anti-PlexA4 mouse monoclonal antibody with or without immunogen [39] overnight at 4 °C, followed by additional incubation with protein G magnetic beads (GE Healthcare) for 1 h at 4 °C. After washing three times with immunoprecipitation buffer, the samples were used for immunoblot analysis with anti-GluA2 mouse monoclonal and anti-PlexA4 rabbit polyclonal antibodies. To produce the mouse monoclonal antibody against PlexA4, the recombinant protein for the Fc-dimerized sema domain of mouse PlexA4 (ref. 39 ) (a.a. 18–588, PlexA4SD-Fc-His6; 50 μg for each shot) emulsified with TiterMax Gold adjuvant (TiterMax USA, Inc.) was injected intraperitoneally into plexinA4 -deficient mice, four to five times at 2-week intervals. Three days after the final booster immunization, spleen cells were collected and fused with myeloma cells P3X63Ag8U1 (P3U1). To confirm the specific interaction between GluA2 and PlexA4, we also employed an anti-PlexAs rabbit polyclonal antibody that recognizes all PlexA families ( Supplementary Fig. 7h ) [14] . HEK293T cells were seeded at 4.0 × 10 5 cells/dish in a 6-cm dish. One day later, the cells were transfected with EGFP-GluA2 or NRP1-Flag together with the full-length, Δect [8] , IPT domain (a.a. 862–1291 of mouse PlexA1 or a.a. 857–1,285 of mouse PlexA4) or ΔIPT (lacking a.a. 857–1,233 of mouse PlexA4) of PlexA1- or PlexA4-Myc expression vector using FuGENE6 transfection reagent (Promega). After 48 h, cells were lysed by immunoprecipitation buffer and then immunoprecipitated with 2 μg of anti-Myc mouse monoclonal antibody (M5546, Sigma). The samples were used for immunoblot analysis of anti-Myc mouse monoclonal (1:5,000 dilution), anti-GFP mouse monoclonal and anti-Flag mouse monoclonal (F1804, 1:5,000 dilution, Sigma) antibodies. Sindbis viral infection The cDNAs of PlexA1-DN [8] , IPT domain of PlexA1 and PlexA4, DN mutant of KIF5A (a.a. 807-1027 of rat KIF5A; KHCCBD) [24] , and dynamitin were subcloned to pSinRep5 (Invitrogen) [50] . The constructs were designed to express the desired protein and EGFP simultaneously, making use of double subgenomic promoter [53] . In utero electroporation Timed-pregnant Wistar rats were anesthetized at E17 with isoflurane and the uterine horns were exposed by way of a laparotomy. To examine the dendritic localization of HA-GluA1 or HA-GluA2, 4 μl of plasmid DNA mixture (EGFP: 0.25 mg ml −1 , HA-GluA1 or GluA2: 0.4 mg ml −1 , PlexA1-IPT or empty vector: 1.35 mg ml −1 ) containing Fast Green was injected through the uterine wall into one of the lateral ventricles of the embryo, and the embryo’s head was electroporated by forceps-type electrodes (BEX), 50 msec electric pulses of 100 V were delivered five times at intervals of 950 ms with a square electroporator (BEX). For the analysis of the distribution of HA-GluAs, male or female pups were perfused intracardially with 4% PFA at P2. The free-floating coronal sections (100 μm) were then immunostained with anti-HA rabbit polyclonal antibody (sc-805, 1:200 dilution, Santa Cruz Biotechnology). They were analysed using a LSM510 with an objective at × 20 (Plan-NEO FLUAR 20 × /50), and the z -axis series of images were superimposed to one image using LSM 5 Image software. To perform quantification, the HA immunofluorescent intensity at the apical side of the perinuclear region (lower half of the cell body outlined by white broken line in Fig. 9c ) and proximal region of apical dendrite (within 15 μm of the initiation point outlined by yellow broken line in Fig. 9c ) were measured by ImageJ software. Mean ratio of HA immunostaining intensity in apical side of perinuclear region and proximal apical dendrite region was then evaluated. To examine the dendritic morphology of CA1 hippocampal neurons, 4 μl of plasmid DNA mixture (EGFP: 0.25 mg ml −1 , PlexA1-IPT or empty vector: 1.75 mg ml −1 ) containing Fast Green was electroporated into rat CA1 hippocampus at E17, and the morphology of apical dendrite visualized by EGFP florescence was observed at P15 of male or female rats. The relative position of the first branch point was quantified. The relative length of the sr was set to 1 (position 0 is the border between sp and sr, position 1 the border between sr and slm) [17] . Analysis of axodendritic transport and growth cone collapse Axonal and dendritic transport of cultured hippocampal neurons were analysed using time-lapse video microscopy [21] . The number of organelles crossing the line drawn on the video monitor was repeatedly counted for 2-min at 1-min intervals. The average number of organelles crossing the line before the application of Sema3A was set to be the base and changes in both anterograde and retrograde transport rate were calculated. Sema3A was applied at the concentration of 2 nM (local application) or 5 nM (bath application). In case of DRG neurons ( Supplementary Fig. 4b ), dissociated DRG neurons were first transfected with EGFP or EGFP-dynamitin expression vector using Amaxa rat neuron nucleofector kit. One day later, the number of organelles crossing the line drawn on the video monitor was counted for 2 min. For growth cone collapse assay of hippocampal neurons, Sema3A was applied and then incubated for 30 min, followed by fixation and staining with Alexa488-phalloidin. To calculate the rate of growth cone collapse, over 50 axonal growth cones were analysed in each experiment, and growth cones that had neither lamellipodia nor filopodia were scored as collapsed growth cones [54] . Immunohistochemical analysis of sema3A -deficient mice The male or female sema3A -deficient mice used in this study had the C57BL/6 genetic background and were genotyped as described [19] . Hydrolysed, paraffin wax-embedded coronal sections (6 μm thick) were used for immunohistochemistry [55] . The following antibodies were used: anti-GluA1 rabbit polyclonal (1:100 dilution), anti-GluA2 mouse monoclonal (1:200 dilution), anti-GRIP1 mouse monoclonal (1:200 dilution) and anti-MAP2 mouse monoclonal (1:200 dilution) antibodies. Slides were analysed using a LSM510 with a × 20 objective lens (Carl Zeiss). Statistical analysis Two-tailed Student’s t -test or one-way analysis of variance (ANOVA) was applied to the data as indicated in the legends. Differences were considered to be significant at P <0.05. All data in text and figures are presented as mean±s.e.m. No statistical test was used to determine sample size. The sample sizes that we chose are similar to those used in previous publications. How to cite this article: Yamashita, N. et al . PlexinA4-dependent retrograde semaphorin3A signalling regulates the dendritic localization of GluA2-containing AMPA receptors. Nat. Commun. 5:3424 doi: 10.1038/ncomms4424 (2014).